Room temperature quantum coherence in a potential molecular qubit The successful development of a quantum computer would change the world, and current internet encryption methods would cease to function. However, no working quantum computer that even begins to rival conventional computers has been developed yet, which is due to the lack of suitable quantum bits. A key characteristic of a quantum bit is the coherence time. Transition metal complexes are very promising quantum bits, owing to their facile surface deposition and their chemical tunability. However, reported quantum coherence times have been unimpressive. Here we report very long quantum coherence times for a transition metal complex of 68 μs at low temperature (qubit figure of merit Q M =3,400) and 1 μs at room temperature, much higher than previously reported values for such systems. We show that this achievement is because of the rigidity of the lattice as well as removal of nuclear spins from the vicinity of the magnetic ion. The essence of a quantum bit is a system that can be put into an arbitrary coherent superposition state of two or more levels. The lifetime of such a superposition state (quantum coherence time) is the time available for the quantum computation. Many remarkable results have been obtained in this area [1] , [2] , [3] , [4] , but suitable qubits for the construction of a real quantum computer that outperforms today’s classical computers have yet to be found. This is partly owing to conflicting requirements: on the one hand, quantum coherence times T M must be orders of magnitude longer than the time for an individual quantum operation. The ratio of these is the qubit figure of merit that should be larger than 10,000 to allow for fault tolerant quantum computing. On the other hand, for some of the most useful quantum algorithms, a great many qubits need to be put into a collective superposition state (entanglement) that requires interqubit interactions. However, interactions of a qubit with its surroundings (including other qubits) are the cause for the decay of the quantum superposition states of the qubits. Electron-spin-based qubits are a good compromise between sufficiently long coherence times and ability to interact with other quantum bits. Coherence times in the millisecond range have been obtained in diamond nitrogen-vacancy (NV) centres [1] . In this material, a substitutional nitrogen atom combines with an adjacent vacancy to form an S =1 species. However, it is challenging to develop many-qubit systems from these materials. Indeed, for example, decreasing the size of the diamond to the nanoscale (which potentially allows stronger interactions with other qubits) drastically decreases the coherence time of the NV centre [5] . Molecular species, such as transition metal complexes, are very promising in this respect, because interqubit interactions can be tailored at will [6] . In addition, molecules can be deposited in regular arrays on surfaces, which is a prerequisite for addressing qubits. Molecular surface self-assembly techniques have reached the stage where the size of the ordered array is essentially determined by the size of the atomically flat plateaus of the substrate [7] . Surprisingly little has been published on quantum coherence times in mononuclear and polynuclear transition metal complexes [8] , [9] . In recent years, especially the quantum coherence in exchange coupled molecular nanomagnets (MNMs) has received much attention [8] , [10] , [11] , [12] , [13] , [14] , [15] , [16] , [17] , [18] , [19] , [20] , [21] , [22] . The often stated advantage of such systems is the presence of additional spin states that can theoretically allow switching of the interqubit coupling [23] . On the other hand, population leakage to these additional spin states is detrimental to qubit performance. Furthermore, their very presence will shorten spin–lattice ( T 1 ) relaxation times [24] , limiting the maximum achievable quantum coherence time [25] . Indeed, quantum coherence times of polynuclear MNMs tend to become immeasurably short above 10 K. This disadvantage has led to renewed interest in mononuclear systems, with quantum coherence being reported at temperatures as high as 80 K (ref. 26 ) It has been shown that in dilute conditions, the (superhyperfine) interaction with nuclear spins that are weakly coupled to the electron spin is the factor that limits the quantum coherence time in MNMs [20] , [27] . Therefore, we have aimed to remove nuclear spins as much as possible from the immediate surroundings of the metal ion that constitutes the qubit. The main magnetic nuclei in typical organic ligands are hydrogens ( 1 H). Carbon (98.9% 12 C), oxygen (99.8% 16 O) and sulfur (99.2% 32,34 S) are virtually nuclear spin free. Nitrogen ( 14 N) possesses a nuclear spin, but its magnetic moment is much weaker. Hence we have used a ligand without hydrogen atoms. Here we report an investigation of quantum coherence in (PPh 4 ) 2 [Cu(mnt) 2 ] ( 1Cu , mnt 2– =maleonitriledithiolate or 1,2-dicyanoethylene-1,2-dithiolate) doped into the diamagnetic isostructural host (PPh 4 ) 2 [Ni(mnt) 2 ] ( 1Ni ). In addition, we investigate the derivative with a deuterated PPh 4 + counter ion. We find quantum coherence times of up to 68 μs at low temperatures, which are among the highest reported for molecular coordination compounds. Importantly, quantum coherence in this system persists up to room temperature with coherence times in the (sub)microsecond range. It is noteworthy that metal dithiolates have been investigated intensively, regarding their conductivity properties, and were shown to be semiconductors or possess metallic or—under pressure—even superconducting properties [28] , [29] , as well as being processable by thin film methods [30] , [31] . Synthesis and sample preparation Compounds 1Cu and 1Ni ( Fig. 1 ) were synthesized by published procedures (see Supplementary Figs 1–5 for characterization data) [32] . The deuterated derivatives 1CuD and 1NiD in which all hydrogen atoms of the PPh 4 + counter ion have been replaced by deuterium were synthesized in the same manner. The salt PPh 4 Br-d20 was synthesized by literature methods [33] . In concentrated conditions, quantum coherence times are limited by intermolecular interactions between electron spins. Hence, to investigate quantum coherence in 1Cu , we prepared powder samples of nominally 0.001 mol percent of 1Cu in diamagnetic 1Ni and 0.01% of 1CuD in 1NiD . These samples ( 1Cu 0.001% and 1Cu 0.01% D ) were investigated by means of pulsed Q-band electron paramagnetic resonance (EPR) spectroscopy ( ν =34–35 GHz). Preliminary measurements showed that at this doping level, electron–electron interactions play no role in the spin dynamics. 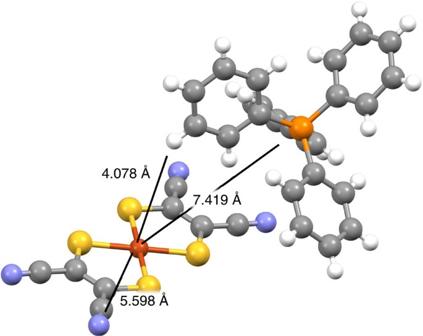Figure 1: Structure of 1Cu. Distances between the metal ion and the nearest nuclei with nonzero spins are indicated in Å. Colours: copper-brown, sulfur-yellow, carbon-grey, nitrogen-blue, phosphorus-orange and hydrogen-white. Figure 1: Structure of 1Cu. Distances between the metal ion and the nearest nuclei with nonzero spins are indicated in Å. Colours: copper-brown, sulfur-yellow, carbon-grey, nitrogen-blue, phosphorus-orange and hydrogen-white. 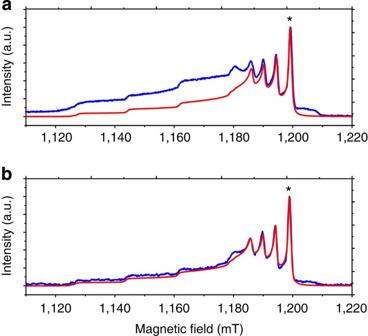Figure 2: ESE-detected Q-band EPR spectra of compound 1Cu0.001%. Experimental results for EPR spectra (blue) recorded atT=7 K (a) andT=120 K (b), and simulation (red) using parameters given in the text. Full size image Electron spin echo-detected EPR spectra Figure 2 shows the electron spin echo (ESE)-detected EPR spectra, recorded by means of the standard Hahn echo sequence with fixed interpulse distances while sweeping the magnetic field ( Supplementary Fig. 6 ). In the low field half of the spectra, four clear widely spaced steps, and in the high-field half four more narrowly spaced peaks can be observed. This spectral shape is common for mononuclear copper(II) complexes and is the result of anisotropic hyperfine coupling of the electron spin to the I =3/2 copper nuclear spin, in combination with an axial g -tensor. Spectral fits ( Fig. 2 ) yielded g || =2.0925±0.0005, g ⊥ =2.0227±0.0005, A || =500±5 MHz, A ⊥ =118±5 MHz. These parameters are quite usual for copper(II) complexes and very comparable to those reported for (NBu 4 ) 2 [Cu(iso-mnt) 2 ] (iso-mnt 2– =iso-maleonitriledithiolate or 1,1-dicyanoethylene-2,2-dithiolate) [34] . The discrepancy between experiment and fit for the 7 K spectrum is not clear to us. It disappears at a temperature of ca. 120 K. Figure 2: ESE-detected Q-band EPR spectra of compound 1Cu 0.001% . Experimental results for EPR spectra (blue) recorded at T =7 K ( a ) and T =120 K ( b ), and simulation (red) using parameters given in the text. Full size image Investigation of quantum coherence The fact that a spin echo is observed at all immediately confirms that quantum coherence is observed in 1Cu 0.001% , even at temperatures as high as 120 K. Hence, we have studied in detail the quantum coherence of 1Cu 0.001% in the temperature range 7–300 K ( Fig. 3 and Supplementary Fig. 7 ), where again we used the Hahn echo sequence, varying the interpulse distance τ . The measurements were performed at the fixed field position given by the asterisk * in Fig. 2 , which corresponds to the transition | m s m I ›=|–1/2, +3/2> to |+1/2, +3/2> in the g ⊥ region. 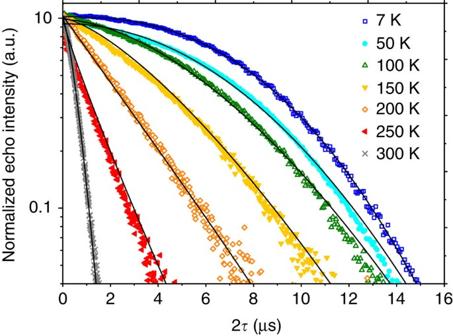Figure 3: Hahn echo decay curves at different temperatures for compound 1Cu0.001%. Integrated echo intensity normalized to the echo intensity immediately after the spectrometer deadtime as a function of delay between initial pulse and echo, at various temperatures as indicated. Solid lines are fits using equation (1), see text. All data could be fitted to stretched exponential decay functions (equation (1)), as is quite common for transition metal systems [9] : Figure 3: Hahn echo decay curves at different temperatures for compound 1Cu 0.001% . Integrated echo intensity normalized to the echo intensity immediately after the spectrometer deadtime as a function of delay between initial pulse and echo, at various temperatures as indicated. Solid lines are fits using equation (1), see text. Full size image where I is the integrated echo intensity, 2 τ is the delay between initial pulse and echo and x is the stretch factor. The factor x ranges between 2 and 3 when the decoherence is dominated by flip-flop processes between nuclear spins (spin diffusion), and is close to 1 when decoherence is dominated by physical motion of the magnetic nuclei [9] . In the latter case the semi-logarithmic plot of I versus 2 τ will be a straight line. Figure 3 demonstrates that this is the case for the coherence time measurements at higher temperatures ( T >150 K). At lower temperatures, x increases and reaches values of almost 2.5 at the lowest investigated temperatures ( Fig. 4 and Supplementary Table 1 ). The coherence time at the lowest measurement temperature ( T =7 K) is 9.23±0.01 μs. This is among the very longest decoherence times ever reported for coordination complexes, and 3.5 times longer than observed for CuPc [26] . To our knowledge, only one paper reports on coherence times that are several times longer, namely for Cr V O(HCA) – and vanadyl ion, both in deuterated H 2 O/glycerol solution [35] . For exchange coupled, polynuclear species, again only one report of a longer coherence time can be found, namely for Cs[Cr 7 NiF 8 (Piv-d9) 16 ], T M =15 μs, albeit at the much lower temperature of 1.5 K (ref. 10 ) The coherence time of 1Cu 0.001% is largely temperature independent up to the very high temperature of ~100 K, beyond which it decreases slowly ( Fig. 4 and Supplementary Table 1 ). Astonishingly, even at room temperature, a respectable coherence time of 600±2 ns was found. From values reported in literature, only vanadyl tetratolylporphyrin comes close [36] . 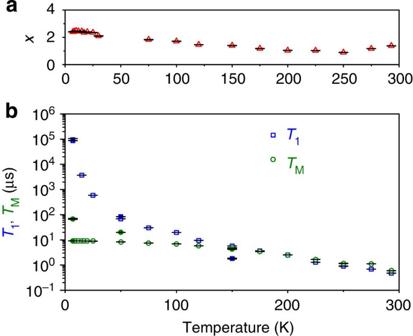Figure 4: Temperature dependence of electron spin relaxation times. (a) Stretch factorxas a function of temperature (1Cu0.001%only). (b) Spin–lattice relaxation (T1) and phase memory time (TM) as a function of temperature. Open symbols belong to1Cu0.001%, filled symbols belong to1Cu0.01%D. Error bars in all panels correspond to the s.d. of the fits. Figure 4: Temperature dependence of electron spin relaxation times. ( a ) Stretch factor x as a function of temperature ( 1Cu 0.001% only). ( b ) Spin–lattice relaxation ( T 1 ) and phase memory time ( T M ) as a function of temperature. Open symbols belong to 1Cu 0.001% , filled symbols belong to 1Cu 0.01% D . Error bars in all panels correspond to the s.d. of the fits. Full size image Our results compare very favourably with those reported for other copper(II) dithiolates, for example, 2% Cu 2+ in (NBu 4 ) 2 [Ni(i-mnt) 2 ] with T M =0.5 μs (ref. 37 ) and a N , N ′-dimethylformamide frozen solution of [Cu(dmit) 2 ] 2– (dmit=1,3-dithiole-2-thione-4,5-dithiolate) with T M =0.52 μs (ref. 38 ) both at low temperatures ( T <25 K). Even in the rather concentrated sample 1Cu1.5%, a coherence time of 3.97±0.05 μs was found at 7 K ( Supplementary Fig. 8 ). Hence, 1Cu clearly outperforms these other copper complexes also in concentrated conditions. This fact shows the importance of small structural details in the design and development of molecular qubits. Hence, 1Cu 0.001% could function as a quantum bit, even at room temperature. To prove that we can perform (simple) coherent spin manipulations, we have carried out nutation measurements at different microwave powers, where Rabi-like oscillations of the echo intensity are clearly observed ( Supplementary Fig. 9 ). Decoherence mechanisms Our earlier investigations on [Fe 4 (acac) 6 (Br-mp) 2 ] (acacH is acetyl acetone and Br-mpH 3 is 2-(bromomethyl)-2-(hydroxymethyl)-1,3-propanediol) revealed a strong correlation between the spin–lattice relaxation time T 1 and the coherence time T M [22] . Therefore, we determined T 1 and its temperature dependence by means of the inversion recovery sequence. The results ( Fig. 4 and Supplementary Fig. 10 ) demonstrate that at high temperatures ( T >120 K), T 1 and T M are indeed essentially the same, suggesting that the latter is determined by the former. In addition, there may be a contribution from nuclear spin motions, for example, librational motions of the phenyl rings of the tetraphenylphosphonium counter ion or of phenyl ring flips [9] . Towards lower temperatures, T 1 increases markedly and reaches T 1 =87.4±0.2 ms at 7 K. Such T 1 times are long, but not unprecedented [9] . The fact that such a wide range of essential temperature independence of T M is found for 1Cu 0.001% is owing to the fact that T 1 is extremely long at low temperatures. T 1 decreases slowly with increasing temperature and only reaches values comparable to T M (10 μs) above 100 K. We attribute the long T 1 to a relatively rigid lattice, as well as the square planar coordination geometry, which is predicted to give rise to longer T 1 times than a tetrahedral geometry [39] . This then suggests that a design criterion for high-temperature molecular qubits is the engineering of a long T 1 . In contrast, at low temperatures, decoherence is dominated by the interaction with nuclear spins. Considering the distances from the crystal structure, the strongest (dipolar) hyperfine coupling is expected to one of the phenyl protons, with A dip,|| =2.5 MHz. The 14 N atom of the dithiolate ligand is much more weakly coupled at A dip,|| =0.10 MHz. Accordingly, we have prepared the derivative of 1Cu with a deuterated PPh 4 + -d 20 counter ion. Pulsed Q-band measurements (on a different, less sensitive pulsed Q-band EPR spectrometer; Fig. 4 , Supplementary Fig. 11 and Supplementary Table 3 ) on the sample 1Cu 0.01% D show an identical quantum coherence time at 150 K (to 1Cu 0.001% ), proving that the results are robust and independent of the used spectrometer. Also, the results are independent of concentration in this range, given that the nominal concentration of the deuterated sample is 10 times higher. Finally, the quantum coherence time is indeed determined by T 1 at this temperature. The T 1 time is slightly shorter, which we attribute to the poor signal to noise at this relatively high temperature. Towards lower temperatures, T M strongly increases, reaching a value of 68±3 μs at 7 K. At lowest temperatures, the decay is biexponential. We attribute the shorter component T M =4.6±0.3 μs to those molecules that possess some electron spin–spin interaction with other molecules, which will statistically occur in a randomly diluted system. The T M value for the slow component is comparable to the abovementioned Cr V O(HCA) – and vanadyl ion in solution. The advantage of 1Cu over these systems are that not only does it have a long coherence time at low temperatures but it also has a quantum coherence time of 1 μs at room temperature (on contrast to Cr V O(HCA) – and vanadyl ion in solution). Second, it is well defined (in contrast to vanadyl ion in solution) and non-toxic (in contrast to carcinogenic chromium(V)) [40] , [41] , important for use in devices. Finally 1Cu belongs to a semiconducting class of compounds (also important for addressing). Taking the ratio of T M and the π/2 pulse length, we arrive at a single qubit figure of merit Q M ≈3,400. We have demonstrated extremely long coherence times both at low (~68 μs) and high temperatures (~1 μs) in 1Cu and 1CuD . This was achieved by removal of weakly coupled nuclear spins and the rigid lattice of the compound. Hence, we have now overcome the first hurdle for the exploitation of molecular compounds as quantum bits in quantum information processing applications. Clearly, there is still scope for improvement by further removing any nuclear spins from the material. In addition, a great deal of work remains to be done on the detailed understanding of the mechanisms behind T 1 and T M , including investigating the frequency and orientation dependences of the relaxation times, as well as the study of hyperfine couplings by means of ENDOR. Finally, optimization of the dithiolate ligand as well as studies on the corresponding vanadyl complexes can be envisioned. All these investigations are now underway. Clearly, material optimization is only the first step on the road to developing a functional quantum computer. We believe that following steps will include tailoring of interqubit interactions [6] , incorporation of photoswitchable linkers to modulate qubit entanglement [42] , surface deposition [26] and implementation of local control, for example, by means of diamond NV centres [43] . Synthesis and sample preparation The compounds 1Cu and 1Ni were prepared according to a literature procedure, and were characterized by infrared, ultraviolet/visible, elemental analysis, SQUID magnetometry and X-ray crystallography ( Supplementary Information ) [32] . Deuterated tetraphenylphosphoniumbromide was synthesized in a pressure cylinder with deuterated starting material according to a literature procedure [33] . The doped powder 1Cu 0.001% was prepared by rapid evaporation of an acetone solution of 1Cu and 1Ni in the correct molar ratio. Samples of 1Cu 0.001% were finely ground, placed into EPR quartz tubes and evacuated overnight. 1Cu 0.01% D was prepared analogously. The tubes were closed with stop cocks (X-band) or by flame-sealing (Q-band). EPR measurements CW X-Band EPR spectra were recorded on a Bruker EMX spectrometer ( ν =9.47 GHz, Stuttgart). Pulsed EPR measurements were performed with a Bruker Elexsys E580 at Q-band ( ν =34 GHz, Frankfurt, 1Cu 0.001% ) and a home-built [44] pulsed Q-band spectrometer ( ν =35 GHz, Stuttgart, 1Cu 0.01% D and 1Cu 1.5% ). Temperatures between 7 and 275 K were obtained with an Oxford Instruments CF935 continuous flow helium cryostat, room temperature measurements were done at ~294 K without external temperature regulation. Typical pulse lengths were 16 ns ( π /2) and 32 ns ( π ) (Frankfurt) and 20 ns ( π /2) and 40 ns ( π ) (Stuttgart). For ESE-detected EPR spectra, the Hahn Echo pulse sequence ( π /2— τ — π — τ —echo) with fixed delay times of τ =140 and 160 ns at 7 and 120 K, respectively, were applied under sweeping the magnetic field. Phase memory times were measured also with Hahn echo sequence, here at a fixed magnetic field under variation of the delay time τ. For measuring spin–lattice-relaxation times, the inversion recovery sequence ( π — T — π /2— τ fix — π — τ fix —echo) with τ fix =140 ns and phase cycling was applied. Nutation measurements were performed with a nutation pulse of variable length followed by a Hahn echo sequence (nutation pulse- τ nut — π /2— τ fix — π — τ fix —echo) with τ nut =400 ns, τ fix =140 ns and different pulse powers. Data analysis and simulation ESE-detected spectra were simulated with EasySpin [45] . Errors of fit parameters ( g and hyperfine values) were estimated by eye. T M relaxation data were normalized to the first measurement point and fitted with Origin, indicated deviations correspond to the standard errors. Phase memory times ( T M ) were extracted from fitting (stretched) exponentials, equation (1), to the Hahn echo decay curves. Experimental data of inversion recovery were fitted with a biexponential function for 7–25 K (fast and slow components) and for higher temperatures mono-exponential fits were applied. How to cite this article: Bader, K. et al. Room temperature quantum coherence in a potential molecular qubit. Nat. Commun. 5:5304 doi: 10.1038/ncomms6304 (2014).